Methylphenidate amplifies the potency and reinforcing effects of amphetamines by increasing dopamine transporter expression Methylphenidate (MPH) is commonly diverted for recreational use, but the neurobiological consequences of exposure to MPH at high, abused doses are not well defined. Here we show that MPH self-administration in rats increases dopamine transporter (DAT) levels and enhances the potency of MPH and amphetamine on dopamine responses and drug-seeking behaviours, without altering cocaine effects. Genetic overexpression of the DAT in mice mimics these effects, confirming that MPH self-administration-induced increases in DAT levels are sufficient to induce the changes. Further, this work outlines a basic mechanism by which increases in DAT levels, regardless of how they occur, are capable of increasing the rewarding and reinforcing effects of select psychostimulant drugs, and suggests that individuals with elevated DAT levels, such as ADHD sufferers, may be more susceptible to the addictive effects of amphetamine-like drugs. Recent epidemiological studies show that rates of illicit drug use have declined in recent years, whereas abuse of prescription drugs, including stimulant medications such as Ritalin, are on the rise [1] . Methylphenidate (MPH), the active compound in Ritalin, is prescribed for attention deficit and hyperactivity disorder (ADHD) and narcolepsy, and is commonly used off-label, with up to 17% of college students reporting abuse of MPH for its cognitive enhancing or euphoric effects [2] . MPH is taken orally, intranasally or intravenously, and is one of the prescribed drugs most diverted onto the illicit market [3] , [4] . MPH abuse occurred at rates comparable to cocaine abuse in the United States in 2008 [5] . However, although there are numerous studies outlining the neurochemical consequences of therapeutic MPH use, there is a paucity of data outlining the neurobiological adaptations that occur during MPH abuse. When taken via the same route of administration, the subjective effects of MPH are indistinguishable from cocaine or amphetamine (AMPH), two commonly abused and highly addictive drugs [6] , [7] . In addition, the behavioural effects of MPH and other psychostimulants are similar. For example, MPH resembles both cocaine and AMPH in extended access self-administration experiments, which result in escalation of intake over sessions, a change thought to model the switch from abuse to addiction [8] , [9] , [10] , [11] . Because of the similar subjective and behavioural profile of MPH compared with highly addictive drugs, it is critically important to ascertain the neurochemical consequences of abuse of MPH. MPH, AMPH and cocaine exert their rewarding and reinforcing effects by inhibiting the dopamine transporter (DAT) and elevating synaptic dopamine levels [12] . In addition, changes in potency at the DAT are predictive of changes in the rewarding effects of these compounds in place preference paradigms [13] . To elucidate the consequences of MPH self-administration on the abuse/addiction potential of psychostimulants, we determined the changes in blocker and releaser potency at the DAT as well as concomitant changes in motivation and drug-seeking behaviours for AMPH, MPH and cocaine. MPH self-administration resulted in increased maximal rates of dopamine uptake mediated by increased DAT levels. Previous work has shown that fluctuations in DAT levels can alter the potency of psychostimulants [14] , although the specific drugs affected and the direction of potency shifts remain equivocal. Here we proposed that MPH self-administration-induced elevations in DAT levels would result in enhanced potency and reinforcing efficacy of releasers and MPH. To test this hypothesis, we used transgenic DAT overexpressing mice (DAT-tg), which have elevated levels of native, non-drug-altered DATs. Using these mice, we elucidated a basic mechanism whereby increased DAT levels drive enhanced potency and motivation to obtain MPH and releaser drugs such as AMPH while leaving the effects of blockers such as cocaine unchanged. The robust enhancement in the potency of releasers, but not blockers, following increases in DAT levels in DAT-tg mice is particularly important as it suggests that individual variations in DAT levels in the human population (for example, ADHD [15] , post-traumatic stress disorder [16] , early-life stress [17] , repeated stressors [18] ) may predict susceptibility to abuse of compounds such as MPH, AMPH and methamphetamine. MPH self-administration increases MPH reinforcement To determine the neurochemical consequences of MPH administration, we allowed rats 6-h access to the most reinforcing dose of MPH (0.56 mg kg −1 per infusion [11] ) on a fixed ratio one (FR1) schedule, with a maximum of 40 injections for 5 consecutive days ( n =11). This resulted in escalation of first-hour intake (one-way analysis of variance (ANOVA); F (4, 10) =20.00, P <0.001) as well as overall rate of intake (one-way ANOVA; F (4, 10) =7.956, P <0.001; Fig. 1a,b ). On an FR1 schedule, it is impossible to differentiate whether increased intake is due to tolerance or increased motivation to take drug; hence, we measured reinforcing efficacy using a progressive ratio (PR) paradigm [19] . We found an increase in breakpoint for MPH (Student’s t -test; t 12 =2.068, P <0.05; Fig. 1c ) following MPH self-administration ( n =7 per group). 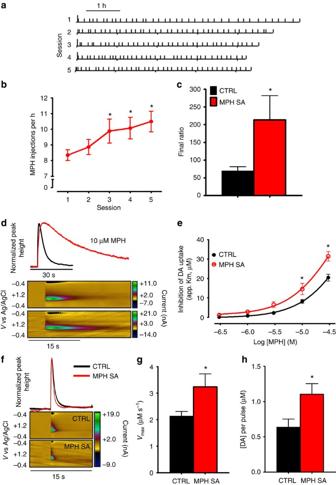Figure 1: MPH self-administration increases dopamine uptake and MPH potency. (a) Self-administration event record from a representative animal. Tick marks represent injections earned. (b) Rate of responding for MPH on a fixed ratio 1 schedule was increased over sessions. Session 1 refers to the first session following acquisition. *P<0.05 versus session 1,n=11 per group, one-way ANOVA. (c) MPH self-administration (red) increased the final ratio during a PR schedule of reinforcement for MPH as compared to minimally trained control animals (CTRL; black). *P<0.05 versus control,n=7 per group, Student’st-test, unpaired. (d,e) MPH self-administration resulted in an increased ability of MPH to inhibit the DAT. *P<0.05 versus control,n=5 control, 6 MPH self-administration, two-way ANOVA. (f–h) MPH self-administration increased the maximal rate of dopamine uptake (Vmax; *P<0.05 versus control,n=31 per group, Student’st-test, unpaired) and stimulated dopamine release ([DA] per pulse) (*P<0.05 versus control, Student’st-test, unpaired). Error bars are reported as mean±s.e.m. DA, dopamine; MPH, methylphenidate; SA, self-administration; CTRL, control. Figure 1: MPH self-administration increases dopamine uptake and MPH potency. ( a ) Self-administration event record from a representative animal. Tick marks represent injections earned. ( b ) Rate of responding for MPH on a fixed ratio 1 schedule was increased over sessions. Session 1 refers to the first session following acquisition. * P <0.05 versus session 1, n =11 per group, one-way ANOVA. ( c ) MPH self-administration (red) increased the final ratio during a PR schedule of reinforcement for MPH as compared to minimally trained control animals (CTRL; black). * P <0.05 versus control, n =7 per group, Student’s t -test, unpaired. ( d , e ) MPH self-administration resulted in an increased ability of MPH to inhibit the DAT. * P <0.05 versus control, n =5 control, 6 MPH self-administration, two-way ANOVA. ( f – h ) MPH self-administration increased the maximal rate of dopamine uptake ( V max ; * P <0.05 versus control, n =31 per group, Student’s t -test, unpaired) and stimulated dopamine release ([DA] per pulse) (* P <0.05 versus control, Student’s t -test, unpaired). Error bars are reported as mean±s.e.m. DA, dopamine; MPH, methylphenidate; SA, self-administration; CTRL, control. Full size image MPH increases MPH potency and MPH-induced dopamine overflow The reinforcing and rewarding effects of many drugs of abuse are related to their ability to elevate dopamine in the nucleus accumbens (NAc) [20] . Although the NAc shell is involved in the acute rewarding effects of drugs and acquisition of self-administration, the NAc core has a critical role in cue-reward learning as well as continued responding for drugs after repeated administration as in the current paradigm [21] , [22] . We found dopamine uptake in the NAc core to be supersensitive to MPH inhibition following MPH self-administration (two-way ANOVA; F (1, 9) =25.11, P <0.05; Fig. 1d,e ; n =5 control, 6 MPH self-administration), which is consistent with our microdialysis data demonstrating increased MPH-induced dopamine overflow in the NAc (two-way ANOVA; F (1, 5) =20.80, P <0.001; Supplementary Fig. S1A ; n =4 control, 5 MPH self-administration). The proposed mechanism for augmented MPH potency is increased DAT levels, which has been suggested to modulate the potency of dopamine releasers [23] . Indeed, after MPH self-administration ( n =31 per group), the maximal rate of dopamine uptake was increased ( V max ; Student’s t -test; t 60 =2.434, P <0.01; Fig. 1g,h ) as was the peak amplitude of stimulated dopamine release ( Fig. 1h ; Student’s t -test; t 24 =2.719, P <0.01). We showed previously that the increase in V max after MPH was due to increased total DAT levels [24] . MPH self-administration increases dopamine releaser potency To further understand the impact of MPH self-administration on psychostimulant potencies, we used voltammetry and microdialysis to examine the ability of a number of DAT blockers and dopamine releasers to enhance dopamine signals in the NAc core. We found that MPH self-administration had no effect on blocker potency, but enhanced the potency of releasers. Thus, the ability of the blockers cocaine ( Fig. 2a,c ; n =5 control, 6 MPH self-administration) and nomifensine ( Fig. 2b,d ; n =5 per group) to inhibit dopamine uptake was unaffected by MPH self-administration. In contrast, the potency of AMPH (two-way ANOVA; F (1, 4) =76.81, P <0.001; Fig. 2e,g ; n =5 per group) and methamphetamine (two-way ANOVA; F (1, 10) =33.51, P <0.001; Fig. 2f,h ; n =7 control, 5 MPH self-administration) was increased. 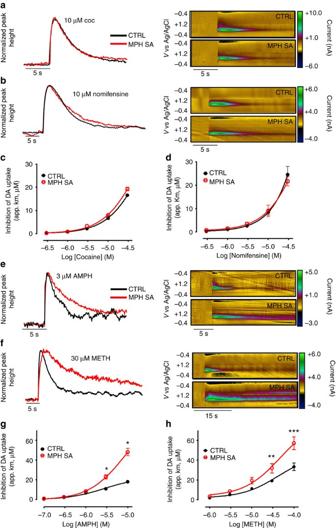Figure 2: MPH self-administration increases the potency of releasers. (a,b) Representative traces showing cocaine- and nomifensine-induced uptake inhibition at the DAT, respectively. Colour plots show the concentration of dopamine (green) over time. The ability of the blockers, (c), cocaine (n=5 control, 6 MPH self-administration), and (d), nomifensine (n=5 per group), to inhibit the DAT following MPH self-administration was unchanged. (e,f) Representative traces showing AMPH- and METH-induced uptake inhibition, respectively. Colour plots show the concentration of dopamine (green) over time. The ability of the releasers (g) AMPH (*P<0.05 versus control,n=5 per group, two-way ANOVA) and, (h), METH (**P<0.01, ***P<0.001 versus control,n=7 control, 5 MPH self-administration, two-way ANOVA) to inhibit the DAT following MPH self-administration was enhanced. Error bars are reported as mean±s.e.m. CTRL, control; DA, dopamine; SA, self-administration; METH, methamphetamine; COC, cocaine; MPH, methylphenidate; AMPH, amphetamine; DAT, dopamine transporter. Figure 2: MPH self-administration increases the potency of releasers. ( a , b ) Representative traces showing cocaine- and nomifensine-induced uptake inhibition at the DAT, respectively. Colour plots show the concentration of dopamine (green) over time. The ability of the blockers, ( c ), cocaine ( n =5 control, 6 MPH self-administration), and ( d ), nomifensine ( n =5 per group), to inhibit the DAT following MPH self-administration was unchanged. ( e,f ) Representative traces showing AMPH- and METH-induced uptake inhibition, respectively. Colour plots show the concentration of dopamine (green) over time. The ability of the releasers ( g ) AMPH (* P <0.05 versus control, n =5 per group, two-way ANOVA) and, ( h ), METH (** P <0.01, *** P <0.001 versus control, n =7 control, 5 MPH self-administration, two-way ANOVA) to inhibit the DAT following MPH self-administration was enhanced. Error bars are reported as mean±s.e.m. CTRL, control; DA, dopamine; SA, self-administration; METH, methamphetamine; COC, cocaine; MPH, methylphenidate; AMPH, amphetamine; DAT, dopamine transporter. Full size image The increase in drug potency for dopamine uptake inhibition by releasers following MPH self-administration was accompanied by increases in drug-induced dopamine overflow as measured using in vivo microdialysis. AMPH (two-way ANOVA; F (1, 5) =11.51, P <0.0001; n =5 control, 6 MPH self-administration; Supplementary Fig. S1B ), but not cocaine ( n =6 per group; Supplementary Fig. S1C ), resulted in increased drug-induced dopamine overflow in the NAc. This confirms that shifts in the ability of releasers to inhibit dopamine uptake correspond to shifts in the ability of releaser to augment extracellular dopamine levels. MPH increases releaser reinforcement and drug-seeking Given the enhanced potency of dopamine releasers, it is possible that these compounds would have increased abuse liability following MPH self-administration. To this end, motivation to take drugs was measured using a ‘threshold’ procedure [25] . The threshold procedure uses a within-session dose response curve, with doses decreasing every 10–15 min, to determine the price (in the form of lever pressing) an animal is willing to pay to receive drug. The maximal price an animal is willing to pay ( P max ) is a measure of the reinforcing efficacy of a compound. After a history of MPH self-administration, there was increased lever responding (two-way ANOVA; F (1, 13) =35.16, P <0.001; Fig. 3a , right) and P max (Student’s t -test; t 14 =2.196, P <0.05; Fig. 3a , left) for MPH ( n =7 control, 8 MPH self-administration). Consistent with the neurochemical data, there was also increased responding (two-way ANOVA, F (1, 11) =51.60, P <0.001; Fig. 3b , right) and P max (Student’s t -test, t 10 =3.136, P <0.01; Fig. 3b , left) for AMPH ( n =7 control, 6 MPH self-administration) but not cocaine ( Fig. 3c ; n =5 control, 6 MPH self-administration). This shows that the increased potency of MPH and AMPH in the NAc is associated with increased drug-seeking behaviour. 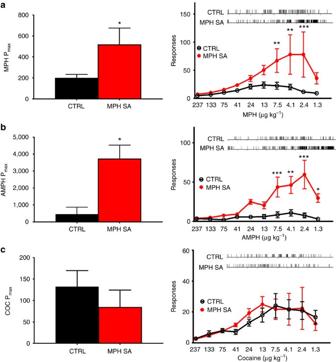Figure 3: MPH self-administration increases the motivation to administer releasers and MPH. (a–c) The maximal price paid (Pmax; left) to administer both MPH (*P<0.05 versus control,n=7 control, 8 MPH self-administration, Student’st-test, unpaired;a, left) and AMPH (*P<0.05 versus control,n=7 control, 6 MPH self-administration, Student’st-test, unpaired;b, left), but not cocaine (n=5 control, 6 MPH self-administration;c, left), was increased following MPH self-administration. The motivation to administer drug for MPH (**P<0.01, ***P<0.001 versus control,n=7 control, 8 MPH self-administration, two-way ANOVA;a, right) and AMPH (*P<0.05, **P<0.01, ***P<0.001 versus control,n=7 control, 6 MPH self-administration, two-way ANOVA;b, right), but not cocaine (n=5 control, 6 MPH self-administration;c, right), was enhanced following MPH self-administration. Error bars are reported as mean±s.e.m. SA, self-administration; COC, cocaine; CTRL, control; MPH, methylphenidate; AMPH, amphetamine. Figure 3: MPH self-administration increases the motivation to administer releasers and MPH. ( a – c ) The maximal price paid ( P max ; left) to administer both MPH (* P <0.05 versus control, n =7 control, 8 MPH self-administration, Student’s t -test, unpaired; a , left) and AMPH (* P <0.05 versus control, n =7 control, 6 MPH self-administration, Student’s t -test, unpaired; b , left), but not cocaine ( n =5 control, 6 MPH self-administration; c , left), was increased following MPH self-administration. The motivation to administer drug for MPH (** P <0.01, *** P <0.001 versus control, n =7 control, 8 MPH self-administration, two-way ANOVA; a , right) and AMPH (* P <0.05, ** P <0.01, *** P <0.001 versus control, n =7 control, 6 MPH self-administration, two-way ANOVA; b , right), but not cocaine ( n =5 control, 6 MPH self-administration; c , right), was enhanced following MPH self-administration. Error bars are reported as mean±s.e.m. SA, self-administration; COC, cocaine; CTRL, control; MPH, methylphenidate; AMPH, amphetamine. Full size image Increased releaser and MPH potency in DAT-tg mice We hypothesized that the increase in releaser and MPH potency was due to the increase in DAT levels and corresponding increase in V max that occurred following MPH self-administration. To test this hypothesis, we used DAT overexpressing mice (DAT-tg) [23] , which have increased levels of native, non-drug-altered DATs. As expected, DAT-tg ( n =16 wild-type (WT), 18 DAT-tg) animals exhibited increased V max (Student’s t -test; t 31 =3.787, P <0.001; Fig. 4a,b ) as well as increased stimulated dopamine release in the NAc core (Student’s t -test; t 31 =2.129, P <0.05; Fig. 4a,c ). We hypothesize that although MPH is categorized as a blocker, it shares some properties of releasers; thus, increases in baseline DAT levels alone would be capable of increasing the neurochemical potency of MPH. In support of our hypothesis and consistent with MPH self-administration results, we showed that increasing DAT levels were sufficient to increase the ability of MPH (two-way ANOVA; F (1, 9) =21.44, P <0.001; n =5 WT, 6 DAT-tg; Fig. 4d ) and AMPH (two-way ANOVA; F (1, 9) =16.05, P <0.001; n =5 WT, 7 DAT-tg; Fig. 4e ), but not cocaine ( n =6 WT, 5 DAT-tg; Fig. 4f ), to inhibit dopamine uptake. Consistent with MPH self-administering animals and voltammetry data, DAT-tg mice had increased MPH- (two-way ANOVA; F (1, 5) =18.53 P <0.001; n =4 per group; Supplementary Fig. S1D ) and AMPH- (F (1, 5) =68.84, P <0.001; n =3 WT, 5 DAT-tg; Supplementary Fig. S1E ), but not cocaine- ( n =4 per group; Supplementary Fig. S1F ), induced dopamine overflow in the NAc. 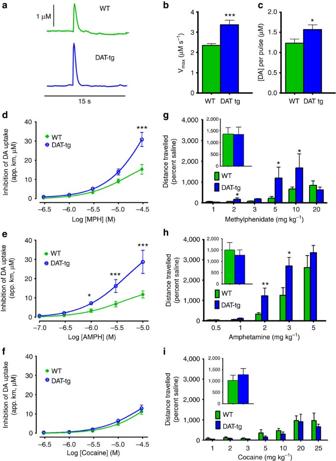Figure 4: Overexpression of DAT increases the behavioural and neurochemical potency of MPH and releasers. (a–c) Rate of dopamine uptake (Vmax; ***P<0.001 versus WT,n=16 WT, 18 DAT-tg, Student’st-test, unpaired) and stimulated dopamine release ([DA] per pulse; *P<0.05 versus WT,n=16 WT, 18 DAT-tg, Student’st-test, unpaired) were increased in DAT overexpressing mice (DAT-tg; blue) relative to WT (green). (d–f) MPH- (***P<0.001 versus control,n=5 WT, 6 DAT-tg, two-way ANOVA) and AMPH- (*P<0.05, ***P<0.001 versus control,n=5 WT, 7 DAT-tg, two-way ANOVA), but not cocaine (6 WT, 5 DAT-t), -induced dopamine uptake inhibition was enhanced in the NAc core of DAT-tg mice as compared with WT. (g–i) Locomotor activating effects of MPH (*P<0.05 versus control,n=6 per group, two-way ANOVA) and AMPH (*P<0.05, **P<0.01 versus control,n=7 WT, 8 DAT-tg, two-way ANOVA), but not cocaine (n=8 WT, 6 DAT-tg), were enhanced in DAT-tg mice. (g–i, insets) Saline-induced locomotion over the 60 min testing period was not different between DAT-tg and WT mice. Error bars are reported as mean±s.e.m. DA, dopamine; MPH, methylphenidate; AMPH, amphetamine;Vmax, maximal rate of dopamine uptake; WT, wild-type. Figure 4: Overexpression of DAT increases the behavioural and neurochemical potency of MPH and releasers. ( a – c ) Rate of dopamine uptake ( V max ; *** P <0.001 versus WT, n =16 WT, 18 DAT-tg, Student’s t -test, unpaired) and stimulated dopamine release ([DA] per pulse; * P <0.05 versus WT, n =16 WT, 18 DAT-tg, Student’s t -test, unpaired) were increased in DAT overexpressing mice (DAT-tg; blue) relative to WT (green). ( d – f ) MPH- (*** P <0.001 versus control, n =5 WT, 6 DAT-tg, two-way ANOVA) and AMPH- (* P <0.05, *** P <0.001 versus control, n =5 WT, 7 DAT-tg, two-way ANOVA), but not cocaine (6 WT, 5 DAT-t), -induced dopamine uptake inhibition was enhanced in the NAc core of DAT-tg mice as compared with WT. ( g – i ) Locomotor activating effects of MPH (* P <0.05 versus control, n =6 per group, two-way ANOVA) and AMPH (* P <0.05, ** P <0.01 versus control, n =7 WT, 8 DAT-tg, two-way ANOVA), but not cocaine ( n =8 WT, 6 DAT-tg), were enhanced in DAT-tg mice. ( g – i , insets) Saline-induced locomotion over the 60 min testing period was not different between DAT-tg and WT mice. Error bars are reported as mean±s.e.m. DA, dopamine; MPH, methylphenidate; AMPH, amphetamine; V max , maximal rate of dopamine uptake; WT, wild-type. Full size image Finally, DAT-tg animals showed increased MPH- (two-way ANOVA; F (1, 10) =4.093, P <0.05; n =6 per group; Fig. 4g ) and AMPH- (two-way ANOVA; F (1, 12) =9.934, P <0.01; n =7 WT, 8 DAT-tg; Fig. 4h ), but not cocaine- ( n =8 WT, 6 DAT-tg; Fig. 4i ), induced locomotion. This further demonstrates that the shifts in neurochemical potency correspond to shifts in the behavioural activating effects of the drug. Oral MPH administration does not alter drug potency Varying the dose and route of administration of a drug can produce variable effects; thus, we aimed to study the effects of oral, therapeutic doses on dopamine kinetics. MPH (5 mg kg −1 ; 2 × day) delivered orally for a period of 14 days ( n =15) resulted in no changes in dopamine kinetics or psychostimulant potencies ( Fig. 5 ). These data suggest that although MPH could enhance the reinforcing efficacy of MPH and releasers when taken via non-oral routes and in larger doses than prescribed, the therapeutic use of MPH does not result in any changes in psychostimulant potencies. 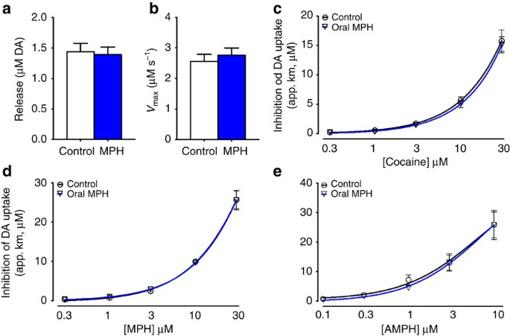Figure 5: Oral MPH administration does not affect dopamine kinetics or the potency of psychostimulants. (a,b) Grouped data from animals treated with oral MPH (5 mg kg−1, 2 × daily, 14 days;n=15 per group; blue) as compared with controls (n=15 per group; white), demonstrating no difference in dopamine system kinetics. (c–e) The potency of cocaine, DA, dopamine; MPH and AMPH was not different between controls (black) and animals with a history of oral MPH self-administration (blue). Error bars are reported as mean±s.e.m. DA, dopamine; MPH, methylphenidate; AMPH, amphetamine. Figure 5: Oral MPH administration does not affect dopamine kinetics or the potency of psychostimulants. ( a , b ) Grouped data from animals treated with oral MPH (5 mg kg −1 , 2 × daily, 14 days; n =15 per group; blue) as compared with controls ( n =15 per group; white), demonstrating no difference in dopamine system kinetics. ( c – e ) The potency of cocaine, DA, dopamine; MPH and AMPH was not different between controls (black) and animals with a history of oral MPH self-administration (blue). Error bars are reported as mean±s.e.m. DA, dopamine; MPH, methylphenidate; AMPH, amphetamine. Full size image Although MPH is often viewed as a safe drug with little addiction potential, emerging evidence indicates that MPH abuse is common and increasing [2] , [3] , [4] . We report here that a rat model of MPH abuse produces profound alterations in dopamine neurotransmission that may enhance vulnerability to addiction. First, we show that MPH self-administration results in escalation of MPH intake and enhances the neurochemical potency and reinforcing effects of MPH and dopamine releasers, but not DAT blockers. Second, increases in DAT levels are sufficient to augment the potency of releasers and MPH, but not blockers. Third, although MPH is traditionally classified as a DAT blocker, it shares some functional properties with releasers. Finally, models of therapeutic use and abuse of MPH have completely different neurochemical consequences. With respect to the first finding, MPH self-administration resulted in escalation of intake over sessions and resulted in enhanced potency of releasers and MPH. The increased rate of intake over sessions was shown to be associated with an increased motivation to administer MPH, as measured by a PR schedule of reinforcement, which is consistent with previous work suggesting that escalation of cocaine intake is due to increased motivation to administer drugs [26] . Because of the fixed injection maximum per session we imposed to reduce variability in intake, animals cannot escalate in total intake. However, first-hour intake was increased, which is a hallmark of traditional escalation [8] , [9] , [10] , [11] , [26] . This first-hour escalation is consistent with work using long-access conditions showing that MPH intake does escalate at a number of doses [11] . Thus, like cocaine and AMPH, MPH intake transitions from low to high levels of intake over time. In addition to enhanced MPH reinforcement, MPH self-administration also resulted in increased motivation to administer AMPH, a dopamine releaser, but not cocaine, a DAT blocker. The increased motivation to administer MPH and AMPH is likely driven by increased MPH and AMPH potency at the DAT and concomitant increases in extracellular dopamine. We found that increased DAT levels, observed following MPH self-administration, were sufficient to elicit the selective increase in MPH and releaser potencies. Indeed, genetic overexpression of the DAT in mice, in the absence of pharmacological intervention, recapitulated the neurochemical and behavioural alterations associated with MPH self-administration. In addition to providing a possible mechanism for the MPH self-administration-induced augmentation of the reinforcing efficacy of releasers, this demonstrates that fluctuations in DAT levels, regardless of how they occur, will change the potency of releaser compounds. Next, we find that DAT level changes alter the potency of dopamine releasers and MPH, but not DAT blockers, despite the general consensus in the field that shifts in cell surface DAT expression lead to inverse shifts in cocaine, but not AMPH, potency. This theory originates from two main sources. The first is that historically, cocaine elevates dopamine in the NAc shell, where DAT levels are low, to a much greater extent than that in the dorsal striatum, where DAT levels are high [27] , [28] . Second, cell culture work shows that DAT overexpression in cells results in a decrease in cocaine potency with no change in the AMPH potency [14] . With respect to the first, the increased potency of cocaine in the shell relative to the caudate has been demonstrated in vivo with microdialysis, and there are a number of factors other than DAT numbers that could influence these results. For example, there are many differences between afferent inputs to caudate and NAc shell, including levels of serotonin and norepinephrine innervations, which are also cocaine targets and influence presynaptic dopamine release. These differences could greatly influence the regional specificity of cocaine effects on dopamine [29] . In addition, previous work using voltammetry in freely moving animals has shown that regional variations in the potency of cocaine are likely attributable to differences in D2 autoreceptor sensitivity in regulating dopamine release, and not differences in DAT levels [30] . With respect to discrepancies with cell culture work, one possibility is that recording endogenous dopamine fluctuations with voltammetry may produce different results than cell culture studies using exogenous [ 3 H]-DA to measure uptake and uptake inhibition [14] . It is possible that [ 3 H]-DA is sequestered into intracellular compartments differently than endogenous DA, and that releaser compounds interact differently with these compartments. Alternatively, it should be noted that many cell culture studies have determined the absolute effects of psychostimulants on dopamine levels, while not necessarily taking into account baseline rates of uptake in the overall effects of these drugs. This is particularly relevant as substantial work has suggested that behavioural outcomes are dependent on a change relative to baseline, not the absolute dopamine levels in isolation [31] , [32] , [33] . Voltammetry determines the effects of the drug while accounting for baseline uptake rates, and this approach correlates well with behavioural outcomes not only in this study but in previous work as well [23] . The DAT-dependent changes in psychostimulant potencies are particularly relevant in clinical treatment settings because disorders such as post-traumatic stress disorder and ADHD are associated with increased DAT levels, ranging from 17 to 70% (refs 15 , 16 , 17 , 18 ). These people could be more sensitive to the neurochemical, behavioural and neurotoxic effects of prescribed AMPH and MPH. In addition, these findings may partially explain the high frequency of drug abuse in untreated ADHD sufferers [34] . Third, this work suggests that MPH is unique in the way in which it interacts with the DAT, and that the characterization of MPH solely as a prototypical DAT blocker may need revision. Indeed, although MPH is considered a DAT blocker, the increased behavioural and neurochemical potency of MPH following both MPH self-administration and DAT overexpression resembles the shift in AMPH’s effects, and not cocaine’s. Moreover, the acute effects of MPH following cocaine self-administration have previously been shown to be similar to releasers and not blockers. For example, Ferris et al. [35] found that cocaine self-administration resulted in DAT tolerance to all blockers, but not releasers or MPH. In addition to the evidence provided by our laboratory, others have shown that, although MPH is not a substrate for the DAT [36] , it functions as a releaser at high concentrations [37] , [38] . In addition, MPH binds to the DAT in a manner that is distinct from prototypical blockers or releasers [39] , [40] , with significant overlap between the binding sites for both cocaine and AMPH. It is possible that although MPH is not transported into the cell, the interaction with the AMPH site results in conformational changes in the DAT, which promote reverse transport in the same way as AMPH. More work is needed to clarify the molecular mechanisms unique to MPH, but our findings suggest that MPH shares some characteristics of both blockers and releasers. Our fourth major finding was that oral administration of low-dose MPH had different neurochemical consequences than self-administration of high-dose MPH. We found that oral administration of low, therapeutic doses had no discernible neurochemical consequences on the dopamine system. This is consistent with other work showing no changes in dopamine kinetics or stimulant potencies following low-dose therapeutic administration of MPH [41] , [42] . This differential effect of MPH at low and high doses may be due to the fact that high-dose MPH substantially elevates dopamine levels in the NAc, whereas low-dose MPH does not [43] , [44] . In addition, changes associated with MPH abuse models may be due to their higher doses and rapid onset, compared with therapeutic administration. In summary, this study shows that MPH self-administration elevates DAT levels and leads to enhanced MPH and dopamine releaser potency. We showed that changes in DAT levels alone were sufficient to alter the potency of psychostimulant releasers and MPH, but not blockers. Thus, MPH is likely increasing DAT levels in individuals that are abusing the drug, which may lead to increased potency for dopamine uptake inhibition, neurotoxicity, and abuse potential for releasers and MPH. In addition, this study demonstrates that MPH potency is altered by transporter fluctuations in a manner that is not significantly different from releasers, although it is not a substrate for the DAT. Thus, we have discovered novel properties of MPH interactions with the DAT, which coincide with novel neuroadaptations following high-dose exposure. Animals Male Sprague–Dawley rats (375–400 g ; Harlan Laboratories, Frederick, MD) were used for all self-administration experiments. Male, C57/Bl6 WT and DAT overexpressing mice were used for locomotor analysis and voltammetry. Animals were maintained according to the National Institutes of Health guidelines in Association for Assessment and Accreditation of Laboratory Animal Care accredited facilities on a 12:12 h light–dark cycle with food and water ad libitum. The experimental protocol was approved by the Institutional Animal Care and Use Committee at Wake Forest School of Medicine. All animals were randomly assigned to experimental groups. There was no blinding done in the current study. Self-administration Male rats (≈ PD 70) were anaesthetized and implanted with chronic indwelling jugular catheters [45] . Following surgery, animals were singly housed, and all sessions took place in the home cage during the active/dark cycle (900–1300 hours). All animals underwent a training paradigm where they were given access to a MPH-paired lever on an FR1 schedule of reinforcement. Training sessions were terminated after a maximum of 20 infusions or 6 h, whichever occurred first. Acquisition occurred when an animal responded for 20 injections for 2 consecutive days. Typically, animals acquired a stable pattern of MPH self-administration within 1–5 days. A small percentage of animals did not acquire self-administration behaviour, but this is typical of self-administration studies. We removed non-acquiring animals from this study. Control animals for PR and threshold self-administration experiments underwent the training paradigm, and then were immediately switched to PR or threshold tests of reinforcing efficacy. We have confirmed that the control group (2 days, 20 MPH injections) is not neurochemically different from naive controls. Treatment animals underwent 5 consecutive days of MPH self-administration. Sessions were 6-h long and were terminated after the animal responded for 40 injections of drug or at the end of the session. The dose of 0.56 mg kg −1 per injection MPH was chosen because it was the dose that produced maximal responding on a dose response curve measuring reinforcing efficacy. It is important to note that this method is different from previously described extended-access paradigms, as animals do not escalate in total intake as an injection limit (40 injections per day) was set to eliminate variability in total consumption of MPH. PR procedure Response requirements were increased through the following ratio progression: 1, 2, 4, 6, 9, 12, 15, 20, 25, 32, 40, 50, 62, 77, 95, 118, 145 and so on. Breakpoints were defined as the number of completed ratios before 1 h elapsed without completion of the next ratio. Data from the MPH self-administration group was compared with a control group (2 days, 20 MPH injections). Differences between groups cannot be due to differences in task learning or experience, as there was no difference in the cocaine threshold task, indicating that there was not an overall increase in task performance with longer experience. Threshold procedure To determine the reinforcing efficacy of psychostimulants, subjects underwent a within-session threshold procedure [25] . Rats were given access to a descending series of 12 unit doses of cocaine, MPH or AMPH (421, 237, 133, 75, 41, 24, 13, 7.5, 4.1, 2.4, 1.3 and 0 μg per injection) on an FR1 schedule during consecutive 10- or 15-min bins within a daily session. As MPH and AMPH are not metabolized as rapidly as cocaine, each bin was 15 min for those compounds, whereas it was 10 min for cocaine. The lever was not retracted at any time during the session. Doses were manipulated by holding the concentration constant and adjusting the pump duration. We switched from a PR procedure because the threshold procedure can assess both drug taking (in the early bins in the session where the dose is high) and drug seeking (within the latter bins where the dose is low and the final bin where animals are responding for saline). Oral MPH administration MPH was administered using an oral dosing procedure in which subjects are trained, in <3 days, to voluntarily consume MPH in a 5-ml volume of 10% sucrose. This procedure results in a pharmacokinetic profile of MPH distribution close to that observed in humans. MPH was administered twice daily (700 and 1400 hours) at a dose of 5 mg kg −1 for 2 weeks (14 days). This dosing regimen takes into account the fact that MPH metabolism is more rapid in rats than in humans and yields blood serum levels near the upper end of the therapeutic range observed in children (5–40 ng ml −1 ). Ex vivo voltammetry Fast scan cyclic voltammetry in brain slices was used to characterize dopamine system kinetics, as well as the ability of psychostimulants to inhibit dopamine uptake in the NAc. Ex vivo voltammetry was chosen because it allows for the accurate assessment of psychostimulant potency by running within-subject concentration response curves for each drug. Voltammetry experiments were conducted during the dark phase of the light cycle, beginning 18 h after commencement of the final self-administration or oral MPH session. A carbon fibre electrode and a stimulating electrode were placed on the surface of the slice in close proximity to each other in the core of the NAc. Endogenous dopamine release was evoked by a single electrical pulse (300 μA, 4 ms, monophasic) applied to the tissue every 5 min. Extracellular dopamine was recorded by applying a triangular waveform (−0.4 to +1.2 to −0.4 V). Once the extracellular dopamine response was stable for three consecutive stimulations, blockers (cocaine and nomifensine), MPH and releasers (AMPH and methamphetamine) were applied to the brain slice. Dopamine current was converted to concentration by electrode calibration with 3 μM dopamine at the end of each experiment. Demon voltammetry and analysis software was used for the analysis [46] . To evaluate the effects of drugs, evoked levels of dopamine were modelled using Michaelis–Menten kinetics as a balance between release and uptake [47] . The Michaelis–Menten modelling provides parameters that describe the amount of dopamine released following stimulation, the maximal rate of dopamine uptake ( V max ) and inhibition of the ability of dopamine to bind to the DAT, or apparent K m . For pre-drug modelling, we followed standard voltammetric modelling procedures by setting the apparent K m parameter to 160 nM based on the affinity of dopamine for the DAT, whereas baseline V max values were allowed to vary as the baseline measure of the rate of dopamine uptake. Following drug application, apparent K m was allowed to vary to account for changes in drug-induced dopamine uptake inhibition while the respective V max value determined for that subject at baseline was held constant. The apparent K m parameter models the amount of dopamine uptake inhibition following a particular dose of drug. Locomotor analysis Locomotor activity was assessed in automated locomotor activity monitors (MedAssociates). Mice were placed into the activity monitor chamber (20 × 20 cm 2 ) for 60 min, and then injected with saline or the drug in 0.1 ml total volume, returned to the chamber and monitored for 60 min after injection. Locomotor activity was measured as horizontal distance covered as a percent of each animal’s saline baseline. Dose response curves were run for each drug. Microdialysis Animals were anaesthetized with ketamine/xylazine, placed in a stereotaxic frame and concentric microdialysis probes (2 mm (rat) or 1 mm (mouse) membrane length; cutoff 6,000 Da; CMA-11, CMA/Microdialysis, Solna, Sweden) were implanted into the NAc core in both rats and mice the day before recording [48] . Appropriate placement of probes was verified by histological examination after the experiments. For rats, microdialysis surgery was performed the day following the final session of MPH self-administration. The day following surgery, probes were perfused with artificial cerebrospinal fluid at 1.0 μl min −1 . Samples were collected every 20 min and analysed for dopamine by HPLC (Bionalytical Systems, Mt. Vernon, IN). Once stable baselines were established, the inlet line was switched to a syringe containing the same artificial cerebrospinal fluid with AMPH (10 μM), MPH (30 μM) or cocaine (30 μM). HPLC A 2 × 50 mm 2 (3 μm particle) reverse-phase column (Luna, Phenomenex, Torrance, CA) was used and the applied potential was +650 mV as referenced to an Ag/AgCl electrode. The mobile phase (75 mM NaH 2 PO 4 , 1.7 mM 1-octanesulfonic acid sodium salt, 100 μl l −1 triethylamine, 25 μM EDTA, 10% acetonitrile v / v , pH=3.0) was pumped at a rate of 170 μl min −1 , with a detection limit for dopamine of 10 pM. Dopamine quantification was achieved by comparing dialysate samples with dopamine standards of known concentration. Statistics Graph Pad Prism (version 5; La Jolla, CA) was used to analyse data sets and compose graphs. Baseline voltammetry, PR and P max data were compared across groups using a two-tailed Student’s t -test. Data obtained from MPH self-administration/DAT-tg animals were subjected to a two-way ANOVA with experimental group and concentration of drug as the factors. TH and locomotor data were subjected to a two-way ANOVA with experimental group and dose as the factors. When significant interactions or main effects were obtained ( P <0.05), differences between groups were tested using Bonferroni post hoc tests. Parametric statistics were used for all analysis. Data met the assumptions of normality, and the variance between groups was similar for all experiments. Power analyses were utilized for every measure to determine the number of animals needed to detect small- to medium-sized effects, with expected effect sizes and s.d. based on previous experiments performed in the laboratory and from published manuscripts. Exclusion of data points only occurred if the points were significant outliers as determined by statistical analysis. How to cite this article: Calipari, E. S. et al. Methylphenidate amplifies the potency and reinforcing effects of amphetamines by increasing dopamine transporter expression. Nat. Commun. 4:2720 doi: 10.1038/ncomms3720 (2013).